FTO-mediated formation ofN6-hydroxymethyladenosine andN6-formyladenosine in mammalian RNA N 6 -methyladenosine is a prevalent internal modification in messenger RNA and non-coding RNA affecting various cellular pathways. Here we report the discovery of two additional modifications, N 6 -hydroxymethyladenosine (hm 6 A) and N 6 -formyladenosine (f 6 A), in mammalian messenger RNA. We show that Fe II - and α-ketoglutarate-dependent fat mass and obesity-associated (FTO) protein oxidize N 6 -methyladenosine to generate N 6 -hydroxymethyladenosine as an intermediate modification, and N 6 -formyladenosine as a further oxidized product. N 6 -hydroxymethyladenosine and N 6 -formyladenosine have half-life times of ~3 h in aqueous solution under physiological relevant conditions, and are present in isolated messenger RNA from human cells as well as mouse tissues. These previously unknown modifications derived from the prevalent N 6 -methyladenosine in messenger RNA, formed through oxidative RNA demethylation, may dynamically modulate RNA–protein interactions to affect gene expression regulation. RNA modifications can affect molecular interaction and structural changes extending beyond local conformation of RNA. Not until recently were some of these modifications discovered to be reversible, dynamic and responsive to cellular stimuli, which suggests that they may participate in cellular regulatory processes [1] , [2] . N 6 -methyladenosine (m 6 A) is a widespread internal modification in messenger RNA (mRNA), which constitutes 1–2% of all adenosine in mRNA [3] . Over 12,000 m 6 A sites in the transcripts of more than 7,000 human genes have been characterized [4] , [5] . Conserved preference of m 6 A around stop codons, in 3′-untranslated region, and within long internal exons have been revealed in both human and mouse cells [4] , [5] . This modification is essential to cell survival and development in eukaryotes, and has a fundamental role in gene expression regulation [6] , [7] . Although the methyltransferase complex is thought to contain METTL3 in mammals [8] , the following have been identified as components of this complex in yeast: Ime4 (yeast m 6 A methyltransferase), Mum2 and Slz1 ( [9] ). We have discovered that the human fat mass and obesity-associated protein FTO catalyses the removal of m 6 A in vitro and in vivo , providing the first example of reversible methylation in RNA [2] . FTO, which was identified in several genome-wide-association studies to be associated with obesity and type II diabetes [10] , [11] , [12] , is a member of the non-haem Fe II /α-ketoglutarate (α-KG)-dependent AlkB family demethylases that mainly catalyse oxidative demethylation of N -alkylated nucleic acid bases [13] , [14] , [15] . We seek to further understand the FTO-mediated oxidative demethylation of m 6 A ( Fig. 1a ) and identify potential new modifications that could be present inside mammalian cells as this family of enzymes exhibits versatile activities [16] . For instance, the recently discovered ten eleven translocation (TET) enzymes that belong to the general family of non-haeme Fe II /α-KG-dependent dioxygenases can perform tandem oxidations [17] , [18] , [19] , [20] . Initially shown to catalyse the oxidation of 5-methylcytosine (5mC) to 5-hydroxymethylcytosine (5hmC) in mammalian genomic DNA [17] , [18] , TET proteins were found to further oxidize 5hmC to 5-formylcytosine (5fC) and 5-carboxylcytosine (5caC) [19] , [20] , [21] . 5hmC levels are highest in the brain extracts and 5hmC is thought to be a new DNA epigenetic marker [22] . The oxidation of 5hmC to 5fC and/or 5caC is a much slower process compared with the oxidation of 5mC to 5hmC ( [20] ). Nevertheless, the continuous oxidation of 5hmC by TET enzymes is essential to an active DNA demethylation pathway, and has important roles in regulating DNA epigenetics [19] , [23] . 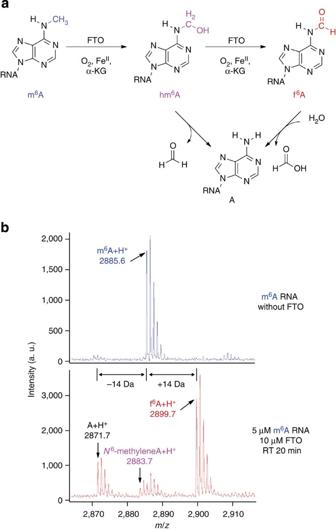Figure 1: Oxidative demethylation of m6A in RNA by FTO. (a) FTO demethylates m6A through oxidization of m6A to hm6A with f6A as a further oxidized product. (b) MALDI-TOF analysis of m6A-RNA after reacting with FTO. An unexpected monoisotopic peak of m6A+14 Da corresponding to f6A was observed after treating a 9mer m6A-RNA oligo (5 μM) with 10 μM of FTO at room temperature (RT) for 20 min. The m6A−2 Da peak represents the dehydration product of the putative hm6A intermediate during MALDI-TOF ionization. Figure 1: Oxidative demethylation of m 6 A in RNA by FTO. ( a ) FTO demethylates m 6 A through oxidization of m 6 A to hm 6 A with f 6 A as a further oxidized product. ( b ) MALDI-TOF analysis of m 6 A-RNA after reacting with FTO. An unexpected monoisotopic peak of m 6 A+14 Da corresponding to f 6 A was observed after treating a 9mer m 6 A-RNA oligo (5 μM) with 10 μM of FTO at room temperature (RT) for 20 min. The m 6 A−2 Da peak represents the dehydration product of the putative hm 6 A intermediate during MALDI-TOF ionization. Full size image Here we show that FTO oxidizes m 6 A to hm 6 A and f 6 A in RNA in a step-wise manner. The observation is further supported by molecular dynamic (MD) simulation, which indicates that FTO can bind to hm 6 A and m 6 A as substrates. We further demonstrate that hm 6 A and f 6 A are relatively stable under physiological conditions and can be detected in polyadenylated RNA isolated from human cells and mouse tissues. These meta-stable intermediates, generated during the course of the FTO-catalysed m 6 A demethylation and discovered for the first time inside mammalian cells, may have significant functional implications. New modifications in the FTO-mediated m 6 A oxidation To investigate the FTO-catalysed demethylation process, we monitored the reaction with high-resolution matrix-assisted laser desorption-ionization time-of-flight mass (MALDI-TOF)/TOF mass spectrometry (MS) to detect hm 6 A, an expected oxidation product of m 6 A in RNA by FTO. Five micromolar of 9mer single-stranded RNA (ssRNA) containing m 6 A was treated with 10 μM of FTO at room temperature for 20 min, and analysed immediately after reaction ( Fig. 1b ). To our surprise, when analysing the monoisotopic peaks, other than the peak of demethylation product (m 6 A−14 Da), we also observed another m 6 A+14 Da peak representing an unknown reaction product ( Fig. 1b ). The putative hm 6 A product has a molecular weight of m 6 A+16 Da, which likely loses a H 2 O moiety (−18 Da) to form N 6 -methyleneadenosine (m 6 A−2 Da) during the process ( Fig. 1b ). We speculated that this unexpected +14 Da peak may correspond to N 6 -formyladenosine (f 6 A) as a result of a tandem oxidation of the m 6 A substrate in a process similar to that of the oxidation of 5mC to 5hmC and 5fC by the TET proteins in the DNA demethylation pathway. As the oxidation of hemiaminal to amide is a rare chemical transformation, and the enzymatic conversion of this process has never been reported, we proceeded to further confirm the identity of this unprecedented species. We reasoned that in previous high-performance liquid chromatography (HPLC) analysis of the digested nucleosides, the basic conditions used during alkaline phosphatase digestion may accelerate the hydrolysis of this reaction product [2] . As FTO showed similar demethylation activity between internal and terminal m 6 A in RNA ( Fig. 1b and Supplementary Fig. S1 ), we synthesized a 9mer ssRNA oligonucleotide with m 6 A incorporated at the 5′ end for further studies. In this case, we could analyse the first nucleoside at the 5′ position with only nuclease P1 digestion to avoid the basic conditions ( Fig. 2a ). Five micromolar of the substrate RNA was treated with 2.5 μM of FTO for 2 or 20 min at room temperature, and the reaction product was digested with nuclease P1 and run through a C18 reverse phase column on HPLC. Two new peaks other than m 6 A and A were observed ( Fig. 2b ). We suspected that the initially generated product was hm 6 A, and the latter product was f 6 A. 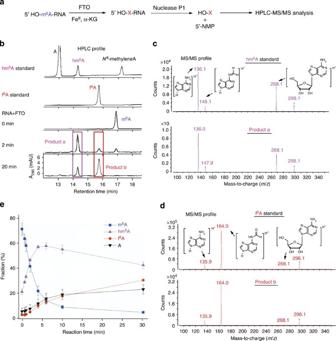Figure 2: Formation of new RNA modifications during oxidative demethylation of m6A in RNA by FTO. (a) A 9mer ssRNA containing a 5′ m6A is used for HPLC-MS/MS analysis. After the RNA is treated with FTO, it is digested by nuclease P1 to release the first base as a nucleoside for further HPLC-MS/MS analysis. The rest of the bases are left as nucleoside 5′-monophosphate (5′-NMP). (b) HPLC analysis of nuclease P1-digested 5′m6A-9mer RNA oligo (5 μM) after treating with FTO. m6A was converted to hm6A and f6A after the treatment with 2.5 μM of FTO for 2 min at room temperature; substantial conversion of hm6A to f6A can be observed in 20 min. These newly formed peaks coelute with hm6A and f6A standards, respectively. The last peak in hm6A standard isN6-methyleneadenosine, a dehydration product that coexists with hm6A. (c,d) Comparison of MS/MS profile of m6A-oxidation products with hm6A and f6A standards. (c) The initial product matches the elution time and MS/MS fragmentation pattern of hm6A. (d) The later-formed product matches the elution time and MS/MS fragmentation pattern of f6A. (e) Kinetic behaviour of the reaction indicates that the formation rate of f6A is slower than the oxidation rate from m6A to hm6A by a factor of 12.3±1.9. Error bars, mean±s.e.m. forn=4 experiments. Figure 2: Formation of new RNA modifications during oxidative demethylation of m 6 A in RNA by FTO. ( a ) A 9mer ssRNA containing a 5′ m 6 A is used for HPLC-MS/MS analysis. After the RNA is treated with FTO, it is digested by nuclease P1 to release the first base as a nucleoside for further HPLC-MS/MS analysis. The rest of the bases are left as nucleoside 5′-monophosphate (5′-NMP). ( b ) HPLC analysis of nuclease P1-digested 5′m 6 A-9mer RNA oligo (5 μM) after treating with FTO. m 6 A was converted to hm 6 A and f 6 A after the treatment with 2.5 μM of FTO for 2 min at room temperature; substantial conversion of hm 6 A to f 6 A can be observed in 20 min. These newly formed peaks coelute with hm 6 A and f 6 A standards, respectively. The last peak in hm 6 A standard is N 6 -methyleneadenosine, a dehydration product that coexists with hm 6 A. ( c , d ) Comparison of MS/MS profile of m 6 A-oxidation products with hm 6 A and f 6 A standards. ( c ) The initial product matches the elution time and MS/MS fragmentation pattern of hm 6 A. ( d ) The later-formed product matches the elution time and MS/MS fragmentation pattern of f 6 A. ( e ) Kinetic behaviour of the reaction indicates that the formation rate of f 6 A is slower than the oxidation rate from m 6 A to hm 6 A by a factor of 12.3±1.9. Error bars, mean±s.e.m. for n =4 experiments. Full size image To confirm the identities of these species, we chemically synthesized hm 6 A and f 6 A standards following reported procedures ( Supplementary Methods and Supplementary Fig. S2 ) [24] , [25] . Briefly, after treating 100 μM of adenosine with 30 mM of formaldehyde at 60 °C for 4 h, hm 6 A was produced, which partially dehydrated to N 6 -methylene-adenosine in equilibrium ( Supplementary Fig. S2a ) [24] . f 6 A could be prepared by treating N , N -dimethylformamidine-protected TBDMS-adenosine with weak acid N -hydroxybenzotriazole (HOBt·H 2 O) in MeOH ( Supplementary Fig. S2b ), followed by deprotection of the TBDMS group [25] . f 6 A is stable in dry organic solvent, and can be further characterized by high-resolution MS, nuclear magnetic resonance (NMR) and ultraviolet-visible (UV–vis) spectra analysis ( Supplementary Figs S3 and S4 ). It has the highest absorbance at 274 nm with ε max (274 nm) =1.83 × 10 4 M −1 cm −1 ( Supplementary Fig. S4 ) in water. The two reaction products coelute with synthesized hm 6 A and f 6 A standards in HPLC ( Fig. 2b ), and have the same MS/MS fragmentation pattern as hm 6 A ( Fig. 2c ) and f 6 A ( Fig. 2d ), respectively, thus confirming their identities. Both hm 6 A and f 6 A decompose to A in aqueous solution, and the hydrolysis processes were accelerated under acidic or basic conditions ( Supplementary Fig. S5 ). To measure the stability of hm 6 A and f 6 A under physiological conditions, hm 6 A- and f 6 A-containing RNA generated by FTO oxidation in situ were digested with nuclease P1, and diluted in buffer solutions mimicking the physiological conditions with Tris–HCl (20 mM, pH 7.4), KCl (140 mM), NaCl (15 mM) and MgCl 2 (1 mM). The solutions were incubated at 37 °C and analysed by HPLC-MS/MS to monitor the degradation process. In the neutral buffered solution, long half-life times of 186±25 min for hm 6 A and 188±18 min for f 6 A were observed, respectively ( Supplementary Fig. S6 ), which are comparable to the average half-life of mRNA in mammalian cells [26] . The relative long life times of hm 6 A and f 6 A under physiological conditions suggest that they are present inside living cells and may have functional roles other than as mere demethylation intermediates. Reaction kinetics of FTO-mediated oxidation To elucidate the kinetic behaviour of the production of hm 6 A and f 6 A, we measured a time-course reaction profile of FTO (2.5 μM) on the same RNA (5 μM) at 37 °C by quantitative LC-MS/MS ( Fig. 2e and Supplementary Fig. S7 ). We found that similar to the oxidation of 5mC to 5hmC and then 5fC by Tet [20] , FTO catalyses the oxidation of hm 6 A to f 6 A at a relatively slower rate compared with the oxidation of m 6 A to hm 6 A ( Fig. 2e ). The kinetic behaviour of this two-step oxidation process suggests a non-processive oxidation pathway, which involves the releasing and rebinding of the hm 6 A intermediate to the FTO active site. Generation of f 6 A will be sensitive to the FTO concentration as the two-step reaction harbours a fast first step and a slow second step; higher local concentrations of FTO will result in the production of more f 6 A. FTO recognizes m 6 A as well as hm 6 A as its substrate To further rationalize our observations, we used MD simulation to model the binding of FTO with m 6 A and hm 6 A. Protein coordinates were retrieved from the crystal structure of FTO- N 3 -methylthymine (m 3 T) complex (PDB ID: 3LFM) [27] ; initial base coordinates were set up in two independent ways. The first approach was to fix the sugar ring position of m 3 T in 3LFM, and mutate m 3 T to N 3 -methylcytosine (m 3 C), m 6 A and hm 6 A. These systems were labelled as FTO-m 3 T-cry, FTO-m 3 C-cry, FTO-m 6 A-cry and FTO-hm 6 A-cry, respectively. The second protocol involves aligning the AlkB–DNA complex crystal structures with FTO based on similarities in protein structure calculated with the Protein Comparison Tool [28] ( Supplementary Figs S8 and S9 ), and then using the coordinates of the lesioned bases from the aligned AlkB complexes [29] . We used PDB file 3O1O to derive the coordinates for m 3 T, 3O1M for m 3 C and 3O1P for εA, respectively; εA was then mutated to m 6 A or hm 6 A. These systems were labelled as FTO-m 3 T-alkb, FTO-m 3 C-alkb, FTO-m 6 A-alkb and FTO-hm 6 A-alkb, respectively ( Supplementary Fig. S10 ). We calculated the binding models of m 6 A ( Supplementary Figs S11 and S12 ) and hm 6 A ( Supplementary Figs S13 and S14 ) in FTO with more than 10-ns MD simulation, in comparison with m 3 T ( Supplementary Figs S15 and S16 ) and m 3 C ( Supplementary Figs S17 and S18 ) (Supporting methods). Similar to m 3 T, both m 6 A ( Fig. 3a ) and hm 6 A ( Fig. 3b ) are stable in the active site in two sets of MD simulations using two initial positions retrieved by two independent methods described above (left panels were calculated using the FTO-m 3 T crystal structure to prepare the initial coordinates of the base; right panels were calculated using aligned AlkB crystal structures to derive the initial base coordinates.). Overlays of these structures with the FTO-m 3 T crystal structure show that N 6 -methyl in m 6 A ( Fig. 3c ) and N 6 -methylene in hm 6 A ( Fig. 3d ) position near the iron centre in the active site of FTO similar to N 3 -methyl in m 3 T in the solved structure [27] . 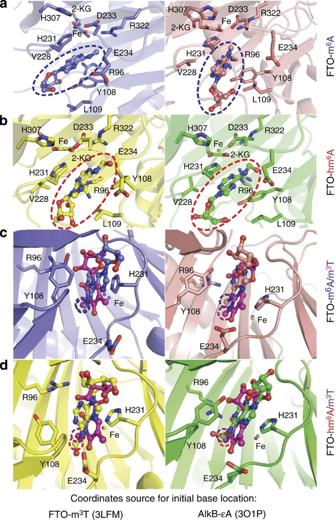Figure 3: Simulated binding mode of m6A and hm6A in FTO after 10 ns of MD simulations. (a) Binding model of FTO-m6A. (b) Binding model of FTO-hm6A. m6A and hm6A is highlighted in dashed blue and red circles. (c) Binding model comparison of m6A overlay with m3T. (d) Binding model comparison of hm6A overlay with m3T. Positions of the targeting methyl in m6A and hm6A are highlighted in dashed blue and red circles, respectively; the targeting methyl in m3T is highlighted in dashed magenta circles. Protein structure is shown in cartoon and active-site residues in sticks. Left panels use the m3T coordinate as in the FTO crystal structure (PDB ID: 3LFM) to prepare the initial location of the base in the FTO simulation through the following steps: fix the sugar ring position in 3LFM and mutate m3T to m3C, m6A, and hm6A, respectively. Right panels use the base coordinates from aligned AlkB crystal structures (PDB ID: 3O1P for εA, and 3O1O for m3T): align FTO and AlkB, take the aligned positions of m3T and εA as the starting point and mutate εA to m6A and hm6A, respectively. As a negative control, m 3 C was observed to be unstable in FTO and dissociated from the active site after 3 ns of simulation ( Supplementary Figs S17 and S18 ), which was likely the result of the positive charge of m 3 C. Figure 3: Simulated binding mode of m 6 A and hm 6 A in FTO after 10 ns of MD simulations. ( a ) Binding model of FTO-m 6 A. ( b ) Binding model of FTO-hm 6 A. m 6 A and hm 6 A is highlighted in dashed blue and red circles. ( c ) Binding model comparison of m 6 A overlay with m 3 T. ( d ) Binding model comparison of hm 6 A overlay with m 3 T. Positions of the targeting methyl in m 6 A and hm 6 A are highlighted in dashed blue and red circles, respectively; the targeting methyl in m 3 T is highlighted in dashed magenta circles. Protein structure is shown in cartoon and active-site residues in sticks. Left panels use the m 3 T coordinate as in the FTO crystal structure (PDB ID: 3LFM) to prepare the initial location of the base in the FTO simulation through the following steps: fix the sugar ring position in 3LFM and mutate m 3 T to m 3 C, m 6 A, and hm 6 A, respectively. Right panels use the base coordinates from aligned AlkB crystal structures (PDB ID: 3O1P for εA, and 3O1O for m 3 T): align FTO and AlkB, take the aligned positions of m 3 T and εA as the starting point and mutate εA to m 6 A and hm 6 A, respectively. Full size image Relative binding free energies of m 6 A and hm 6 A to FTO were also calculated by alchemical free-energy simulations [30] ( Supplementary Methods , Supplementary Figs S19 and S20 ). All independent simulations predicted a slightly stronger binding (ranging from 0.4 to 2.8 kcal mol −1 ) for hm 6 A over m 6 A ( Supplementary Table S1 ). These data support our observation of hm 6 A as a substrate for FTO, and suggest a similar oxidation model of m 6 A to hm 6 A for hm 6 A to f 6 A, in agreement with the kinetic behaviour of the oxidation reaction and a proposed non-processive tandem oxidation reaction pathway. Detection of hm 6 A and f 6 A in human and mouse mRNA To confirm the existence of these new modifications in vivo , we optimized RNA digestion conditions using RNase T1 followed by nuclease P1 at neutral pH, in which both hm 6 A and f 6 A are relatively stable. RNase T1 cleaves the phosphodiester bond after G, and exposes the following nucleotide with a free 5′-OH. Nuclease P1 releases this nucleotide for subsequent HPLC separation ( Fig. 4a ). Although m 6 A shows a preference in the consensus sequence of (G/A/U)(G>A)m 6 AC(U>A>C) [4] , [5] , this method can analyse hm 6 A and f 6 A present in this consensus sequence after G. Applying this method we analysed the isolated poly(A)-RNA from cultured HeLa cells and mouse liver tissues by LC-MS/MS. We observed peaks with the same elution times at the MS/MS detection channel of hm 6 A (298.1 fragmented to 136.0, Fig. 4b ). 6 A (296.1 fragmented to 164.1, Fig. 4c ), respectively. We subsequently followed the f 6 A peak, which is more stable than hm 6 A. f 6 A in mouse liver decreased significantly upon incubating at room temperature overnight ( Supplementary Fig. S21 ), similar to that observed with the f 6 A standard. Therefore, we confirmed the presence of hm 6 A and f 6 A in poly(A)-RNA in vivo . The concentration of the isolated f 6 A (a large portion of f 6 A may have decomposed during the isolation process) was estimated to be at least 0.5–1% of the total m 6 A ( Supplementary Fig. S22 ). A similar amount of hm 6 A appears to also exist in vivo based on our results. Therefore, taking account of decomposition during isolation a noticeable portion of mRNA should carry either hm 6 A or f 6 A at any given time inside cells. 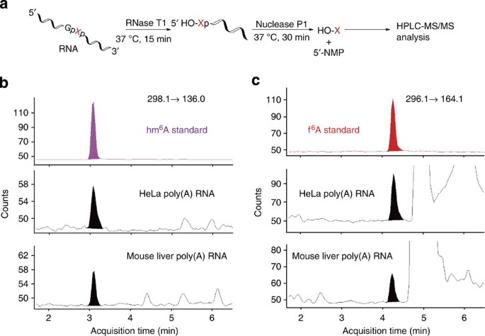Figure 4: Presence of hm6A and f6A in mammalian mRNA. (a) Detection strategy: RNA is first digested with RNase T1 to expose the 5′ OH group of the base after G. Subsequent nuclease P1 digestion releases the first base as nucleoside, and the rest of the bases as nucleoside 5′-monophosphate (5′-NMP). (b,c) LC-MS/MS analysis of digested mRNA isolated from HeLa cell and mouse liver samples showing the presence of hm6A (b, 298.1→136.0, 3.1 min) and f6A (c, 296.1→164.1, 4.2 min). Figure 4: Presence of hm 6 A and f 6 A in mammalian mRNA. ( a ) Detection strategy: RNA is first digested with RNase T1 to expose the 5′ OH group of the base after G. Subsequent nuclease P1 digestion releases the first base as nucleoside, and the rest of the bases as nucleoside 5′-monophosphate (5′-NMP). ( b , c ) LC-MS/MS analysis of digested mRNA isolated from HeLa cell and mouse liver samples showing the presence of hm 6 A ( b , 298.1→136.0, 3.1 min) and f 6 A ( c , 296.1→164.1, 4.2 min). Full size image hm 6 A and f 6 A may modulate RNA–protein interactions As the oxidation of 5mC to 5hmC and then 5fC in DNA hinders binding to methyl-CpG-binding (MBD) proteins [31] , we envisioned that the extra oxygen group on hm 6 A and f 6 A may hinder their interaction with m 6 A-binding proteins. Recently, YTHDF2 protein has been implicated as a potential m 6 A-RNA-binding protein [4] . To evaluate its binding affinity to these RNA modifications, we cloned and expressed a GST-tagged YTHDF2 protein. The binding affinities of YTHDF2 to RNA containing hm 6 A or f 6 A, generated in situ by FTO-mediated oxidation, were measured and compared with those with m 6 A or A using electrophoretic mobility shift assay ( Supplementary Fig. S23 ). About 70% of hm 6 A ( Supplementary Fig. S24 ) and 60% of f 6 A ( Supplementary Fig. S25 ) were estimated to be present in the electrophoretic mobility shift assay assay, respectively, as shown by LC-MS/MS analysis of an unlabelled 9mer RNA that contained 5′-m 6 A treated using the same procedure. We found that the YTHDF2 protein preferentially binds to m 6 A-RNA, while the binding affinities of YTHDF2 to hm 6 A or f 6 A were attenuated to a level similar to A ( Supplementary Fig. S23 ). We show here that hm 6 A and f 6 A are new RNA modifications in mammalian cells, and that FTO can catalyse the formation of these modifications. The AlkB protein has been shown to oxidize m 6 A to hm 6 A as an oxidation intermediate in vitro with no further oxidation of hm 6 A observed [32] . FTO shows the unique activity of performing a second oxidation on the meta-stable hm 6 A to form an unprecedented f 6 A. Compared with other hemiaminal intermediates, hm 6 A is relatively stable because of the electron-rich nature of the exocyclic N 6 nitrogen of adenosine when compared with endocyclic positions, which allows for further oxidation to f 6 A. Although more than 100 RNA modifications have been discovered, the chemical diversity of the modifications is relatively limited. Recent application of more sensitive analytical methods leads to the discovery of RNA modifications with novel functional groups, such as geranylated RNA in bacteria [33] . The discovery of hydroxymethylated and formylated adenosines in mRNA here further expands the repertoire of chemical diversity of RNA modifications. As m 6 A has not only been detected in mRNA but also long non-coding RNA, it is possible that hm 6 A and f 6 A, which are derived from m 6 A, may also exist in long non-coding RNAs. FTO exhibits a relatively high activity towards m 6 A on ssRNA, but lower activity towards m 6 A in stem–loop structures and negligible activity against m 6 A on double-stranded RNA in vitro [2] . The in vivo activity could be affected by the secondary structure of the RNA and cellular machineries that recruit FTO to specific RNA substrates. FTO, ALKBH5 (the second RNA demethylase recently discovered by us [34] ), and the methyltransferase components orchestrate together to determine the modification status of mRNA. As FTO and ALKBH5 are partially localized in nuclear speckles [2] , [34] , in which the methyltransferase complex resides, the demethylated RNA could be remethylated by the methyltransferase in a direct reversible model. In contrast, the temporary existence of the hydroxymethyl and the formyl group on the N 6 position of adenosine may represent a delayed reversible model, in which an additional diffusion/export step may be incorporated and coupled with the ‘slow’ hydrolysis step ( Fig. 5 ). Therefore, these meta-stable intermediates could provide a time-window for the oxidized RNA to diffuse or be exported out of the nuclear speckles, thus eliminating the possibility of remethylation by the methyltransferase complex at the same loci in vivo ( Fig. 5 ). It is also interesting to speculate about other functional roles of hm 6 A and f 6 A because they are not recognized by m 6 A-binding proteins such as YTHDF2. They could serve as another modification marker to recruit different sets of RNA-binding proteins, and differentially regulate the subsequent RNA-related pathways ( Fig. 5 ), or they could serve as markers for nascent RNAs taking advantage of their intrinsic degradation kinetics. It is also interesting to note that the FTO-mediated formation of hm 6 A and f 6 A is similar to the TET-mediated oxidation of 5mC to 5fC and 5caC in DNA [19] , [20] , [21] . Although hm 6 A and f 6 A are inherently unstable, it is possible that additional protein factors could be involved to promote the FTO-mediated demethylation of m 6 A by catalysing the hydrolysis of hm 6 A and f 6 A; on the other hand, hm 6 A and f 6 A can also be stabilized when buried in a hydrophobic environment of their potential binding proteins. Further studies to explore the potential functions of these two modifications are required in the future to address these hypotheses. 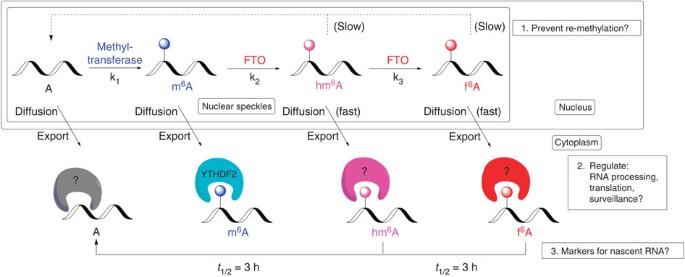Figure 5: A proposed model of dynamic regulation of RNA modifications by FTO. Instead of direct demethylation, a delayed model is proposed for FTO, which possesses different kinetic behaviour to accommodate additional diffusion/export process and avoid direct remethylation. The nascent transcribed RNA is partially methylated by methyltransferase to m6A. m6A is converted to hm6A in regions with low FTO levels, and to f6A in regions with high FTO levels. Demethylated A is produced after the decomposition of hm6A and f6A, which is slower than the diffusion/export process, and which may help to avoid the remethylation by methyltransferase at the nuclear speckles. When RNA is processed and exported to the cytoplasm, different modifications on mRNA can potentially recruit or repel different protein factors, which could affect the metabolisms of mRNA. hm6A and f6A in RNA will eventually be hydrolysed to A; these modifications may also serve as markers for nascent RNA. Figure 5: A proposed model of dynamic regulation of RNA modifications by FTO. Instead of direct demethylation, a delayed model is proposed for FTO, which possesses different kinetic behaviour to accommodate additional diffusion/export process and avoid direct remethylation. The nascent transcribed RNA is partially methylated by methyltransferase to m 6 A. m 6 A is converted to hm 6 A in regions with low FTO levels, and to f 6 A in regions with high FTO levels. Demethylated A is produced after the decomposition of hm 6 A and f 6 A, which is slower than the diffusion/export process, and which may help to avoid the remethylation by methyltransferase at the nuclear speckles. When RNA is processed and exported to the cytoplasm, different modifications on mRNA can potentially recruit or repel different protein factors, which could affect the metabolisms of mRNA. hm 6 A and f 6 A in RNA will eventually be hydrolysed to A; these modifications may also serve as markers for nascent RNA. Full size image In summary, the identification of hm 6 A and f 6 A in cellular mRNA shows that additional modifications can be installed onto the N 6 -position of adenosine, which impact protein–RNA interaction to perhaps provide further dynamical tuning of the function/status of mRNA. Therefore, the discovery of these additional modifications on mRNA presents many intriguing questions and new biology to be explored. General materials and methods Complementary DNA clone of full-length human FTO and YTHDF2 was purchased from Open Biosystems. All primers were purchased from Eurofins MWG Operon. All RNase-free solutions were prepared from DEPC-treated MilliQ-water. Synthesis and characterization of synthetic f 6 A standard Detailed description of the synthesis of f 6 A standard can be found in the Supplementary Methods . The f 6 A standard was characterized by HPLC-QQQ-MS/MS, high-resolution mass spectra, UV–vis spectra, and both 1 H and 13 C NMR ( Supplementary Figs S2–S4 ). Characterization data of f 6 A: 1 H NMR (DMSO-d 6 , 500 MHz) δ 11.395 (br, 1H), 9.953 (s, 1H), 8.766 (s, 1H), 8.617 (s, 1H), 6.034 (d, J =5.5 Hz, 1H), 5.574 (d, J =6.0 Hz, 1H), 5.278 (d, J =5.0 Hz, 1H), 5.185 (t, J =5.5 Hz, 1H), 4.625 (dd, J =5.5 Hz, 5.5 Hz, 1H), 4.202 (dd, J =5.0 Hz, 4.0 Hz, 1H), 4.001 (dd, J =3.5 Hz, 4.0 Hz, 1H) 3.713 (m, 1H), 3.607 (m, 1H) p.p.m. ; 13 C NMR (DMSO-d 6 , 125 MHz) 165.193, 152.995, 152.649, 150.665, 144.237, 122.245, 88.690, 86.697, 74.769, 71.239, 62.204 p.p.m.. UV/Vis: λ max 274 nm, ε (260 nm) =1.30 × 10 4 M −1 cm −1 , ε max(274 nm) =1.83 × 10 4 M −1 cm −1 , LC-QQQ-MS/MS (Positive): [M+H] + =296.1, [Base+H] + =164.0, high-resolution MS ( m / z ) for C 11 H 13 N 5 O 5: [M+H] + =296.0995 (calculated), 296.1009 (found). Synthesis of m 6 A-RNA oligo m 6 A phosphoramidite ( N 6 -methyl-5′- O -(4,4′-dimethoxytrityl)-2′- O - t -butyldimethylsilyl adenosine 3′- O -(2-cyanoethyl- N,N -diisopropyl)phosphoramidite) was synthesized according to a previously reported procedure [35] . RNA oligo containing m 6 A was synthesized using m 6 A RNA phosphoramidite and standard RNA phosphoramidite (Glen Research) under ultra-mild conditions using 1H-tetrazole as activator reagent in an Expedite Nucleic Acid Synthesis System (PerSeptive Biosystems) with DMT-ON protocol. The oligo was cleaved from the beads and purified in a Glen-Pak RNA purification cartridge (Glen Research) according to the standard protocol provided by the manufacturer. The quality and purity of synthesized RNA was monitored by high-resolution MALDI-TOF-MS. Synthesized RNA sequence: RNA oligo with internal m 6 A: CUGGm 6 ACUGG, RNA oligo with 5′ m 6 A: m 6 ACUGACUAG. Biochemistry assay of FTO activity in vitro N-terminal his-tagged truncated human FTO protein (his 6 -FTO-NΔ31) was expressed and purified as previously reported [27] . The demethylation activity assay was performed in 20–100 μl of reaction mixture containing RNA with m 6 A, FTO, 75 μM of (NH 4 ) 2 Fe(SO 4 ) 2 ·6H 2 O, 300 μM of α-KG, 2 mM of L -ascorbic acid, 150 mM of KCl and 50 mM of HEPES buffer (pH 7.0). The reaction was incubated at room temperature or 37 °C, and quenched by the addition of 1 mM of EDTA. The reaction was then frozen in liquid N 2 immediately, and thawed only before analysis was performed. For HPLC or HPLC-MS/MS analysis, the reaction mixture was digested by 1 U of nuclease P1 at 37 °C for 15 min. HPLC analysis was performed on a HPLC system equipped with an Agilent Eclipse XDB-C18 analysis column (150 × 4.6 mm) eluted with buffer A (50 mM ammonium acetate in H 2 O) and buffer B (50 mM ammonium acetate in 60% of acetonitrile in H 2 O) with a flow rate of 1 ml min −1 at room temperature. The detection wavelength was set at 260 nm and 280 nm. HPLC-MS/MS was carried out by reverse-phase ultra-performance liquid chromatography on an Agilent ZORBAX Eclipse XDB-C18 column (Rapid Resolution HT, 50 × 2.1 mm) eluted with buffer A (0.1% formic acid in H 2 O) and buffer B (0.1% formic acid in methanol) with a flow rate of 0.5 ml min −1 at 35 °C, with online mass spectrometry detection using Agilent 6410 triple-quadrupole (QQQ) LC mass spectrometer in multiple reaction monitoring–positive electrospray ionization mode. The nucleosides were quantified using the nucleoside to base ion mass transitions of 282.1 to 150.1 (m 6 A), 268.0 to 136.0 (A), 296.1 to 164.1 (f 6 A) and 198.1 to 136.1 (hm 6 A). Quantification was performed by comparison with the standard curve obtained from synthetic nucleoside standards running at the same batch of samples. MALDI-TOF-MS analysis of RNA oligo The RNA/FTO reaction solution was first desalted by mixing with 50 μl of ammonium-charged AG 50 W-X8 Cation Exchange Resins (Bio-Rad). One microlitre of the desalted solution was then mixed with an equal amount of MALDI matrix, which was composed by 9:1 (v:v) ratio of 2′,4′,6′-trihydroxyacetophenone (THAP, 10 mg ml −1 in 50% CH 3 CN/H 2 O):diammonium citrate (50 mg ml −1 in H 2 O). The mixture was then spotted on a MALDI sample plate, dried under vacuum and analysed by a Bruker Ultraflextreme MALDI-TOF-TOF Mass Spectrometers in reflector, positive mode. Analysis of hm 6 A and f 6 A in mRNA using HPLC-MS/MS Total RNA was isolated from cultured cell or mouse tissues using TRIzol reagent according to the manufacture procedure. mRNA was then isolated with biotin-oligo(dT) and streptavidin beads from Promega, following a modified procedure, which eliminated all heating steps. Eight micrograms of mRNA was digested with RNase T1 in 20 μl for 15 min at 37 °C, followed by nuclease P1 (1 U) for 30 min at 37 °C. The solution was diluted five times, and 20 μl of the solution was analysed by HPLC-QQQ-MS/MS. The nucleosides were quantified using the nucleoside to base ion mass transitions of 282.1 to 150.1 (m 6 A), 268.0 to 136.0 (A), 296.1 to 164.1 (f 6 A) and 198.1 to 136.1 (hm 6 A) in multiple reaction monitoring–positive electrospray ionization mode. MD and alchemical free-energy simulations The initial coordinates were taken from the crystal structure of FTO bound with Fe 2+ , N -oxalylglycine and m 3 T (PDB ID: 3LFM). We replaced the N -oxalylglycine (antagonist of FTO) with the active cofactor α-KG. The coordinates of the modified bases were generated in two different ways, and two independent sets of simulations were carried out accordingly. The first approach was to fix the sugar ring position of m 3 T in 3LFM, and then mutate the original m 3 T to m 3 C, m 6 A or hm 6 A, respectively. These systems were labelled as FTO-m 3 T-cry, FTO-m 3 C-cry, FTO-m 6 A-cry and FTO-hm 6 A-cry, respectively. The second protocol was to align the AlkB–DNA complex crystal structures with FTO based on three-dimensional protein structure similarity calculated with the Protein Comparison Tool and then take the coordinates of the modified bases from the aligned AlkB complexes. We used PDB file 3O1O to derive the coordinates for m 3 T, 3O1M for m 3 C and 3O1P for εA; εA was then mutated to m 6 A or hm 6 A. These systems were labelled as FTO-m 3 T-alkb, FTO-m 3 C-alkb, FTO-m 6 A-alkb and FTO-hm 6 A-alkb, respectively. Detailed procedure for MD simulation set-up and alchemical free-energy simulations for relative binding affinities are provided in Supplementary Methods . How to cite this article: Fu, Y. et al . FTO-Mediated Formation of N 6 -hydroxymethyladenosine and N 6 -formyladenosine in mammalian RNA. Nat. Commun. 4:1798 doi: 10.1038/ncomms2822 (2013).